A new protein complex promoting the assembly of Rad51 filaments During homologous recombination, eukaryotic RecA homologue Rad51 assembles into a nucleoprotein filament on single-stranded DNA to catalyse homologous pairing and DNA-strand exchange with a homologous template. Rad51 nucleoprotein filaments are highly dynamic and regulated via the coordinated actions of various accessory proteins including Rad51 mediators. Here, we identify a new Rad51 mediator complex. The PCSS complex, comprising budding yeast Psy3, Csm2, Shu1 and Shu2 proteins, binds to recombination sites and is required for Rad51 assembly and function during meiosis. Within the hetero-tetramer, Psy3-Csm2 constitutes a core sub-complex with DNA-binding activity. In vitro , purified Psy3-Csm2 stabilizes the Rad51–single-stranded DNA complex independently of nucleotide cofactor. The mechanism of Rad51 stabilization is inferred by our high-resolution crystal structure, which reveals Psy3-Csm2 to be a structural mimic of the Rad51-dimer, a fundamental unit of the Rad51-filament. Together, these results reveal a novel molecular mechanism for this class of Rad51-mediators, which includes the human Rad51 paralogues. Homologous recombination (HR) has a key role in the maintenance of genome stability, but also in generating genetic diversity. Recognition and exchange between two homologous DNAs are a key step for HR and are catalysed by RecA/Rad51 family proteins. In eukaryotes, Rad51 oligomerizes onto single-stranded DNA (ssDNA) to form a right-handed helical filament [1] , [2] . This Rad51 nucleoprotein filament is an essential protein machine for homology search and strand exchange [3] , [4] . The assembly and disassembly of Rad51 filaments is highly dynamic and regulated by various positive and negative factors. In vivo , Rad51 filament assembly necessitates the displacement of RPA (replication protein-A) from ssDNA. Rad51-loading on RPA-coated ssDNAs is aided by a class of proteins termed Rad51 mediators, which includes Rad52 (ref. 5 ), Rad55–57 (Rad51 paralogues) [6] , Sfr1-Swi5 (ref. 7 ) and the Brca2–Dss1 complex [8] , [9] . Each mediator is likely to facilitate Rad51 assembly via a different mechanism. However, it remains unclear how the different Rad51 mediators facilitate and coordinate formation of Rad51 filaments. In Saccharomyces cerevisiae , mutations in a group of genes, PSY3 , CSM2 , SHU1 and SHU2, were identified as suppressors of the slow growth phenotype of a top3 (topoisomerase III) mutant [10] . These mutants also show genome instability in both mitosis and meiosis [11] , [12] , [13] . Recent studies reveal genetic interactions between RAD51 and PSY3/CSM2/SHU1/SHU2 and show that they are involved in Rad51-dependent DNA repair during S-phase [14] , [15] . Moreover, genome-wide analysis showed that these mutations are classified into a single epistasis group [16] . However, exactly how the Psy3, Csm2, Shu1 and Shu2 proteins facilitate DNA repair remains enigmatic. In this study, we show that Psy3, Csm2, Shu1 and Shu2 form a stable hetero-tetramer, which we refer the PCSS complex (a.k.a. the Shu complex), with Psy3-Csm2 as the core dimer. In meiosis, the PCSS complex binds to sites of DNA double-strand breaks (DSBs) and has a critical role in meiotic recombination. Importantly, the PCSS complex is required for formation of Rad51 complexes on meiotic chromosomes, implying a role in mediating assembly of Rad51 nucleoprotein filaments. In vitro , Psy3-Csm2 binds DNA and stabilizes the Rad51–ssDNA complex independently of nucleotide cofactor by forming a ternary complex. Finally, solution of the Psy3-Csm2 crystal structure reveals that Psy3-Csm2 is structurally very similar to a Rad51-dimer, which is the basic protomer of a Rad51 filament. Structure modelling predicts that Psy3-Csm2 dimer binds to the end of Rad51 filament, and in this way may stabilize the filament. This idea was confirmed by analysis of an interface mutant of Csm2 to Rad51. We conclude that the PCSS complex is a new Rad51 mediator that promotes Rad51 filament formation by mimicking the Rad51 structure. Psy3, Csm2, Shu1 and Shu2 form a stable complex in vivo Previous studies demonstrated two-hybrid interactions among the Psy3, Csm2, Shu1 and Shu2 proteins [10] , suggesting that they form a complex. To test this idea, 3FLAG-tagged Shu1 was affinity-purified from meiotic and mitotic cell extracts. Only three bands specific to Shu1-3FLAG were detected by silver staining, occurring in a 1:2:1 ratio ( Fig. 1a ). Western analysis in wild-type and mutant strains revealed that the lower band corresponds to Shu1-3FLAG, the middle band contains both Csm2 and Shu2, and the largest band contains Psy3 (middle panel of Supplementary Fig. S1a,1b ). These results were confirmed by affinity tagging Psy3 and Shu2 (right panel of Supplementary Fig. S1a ; lanes 1, 3 in Supplementary Fig. S1c ). Gel filtration analysis of the purified complex reveals a single peak that elutes around 100 kDa and contains Psy3, Csm2 and Shu1 (and by extension, Shu2; Fig. 1b ). This is consistent with the calculated molecular weight of 96 kDa for a tetramer species containing all four proteins. These data indicate that Psy3, Csm2, Shu1 and Shu2 form a hetero-tetramer in vivo . Hereafter, we refer this complex as the PCSS (Psy3-Csm2-Shu1-Shu2). Importantly, affinity-purified PCSS does not contain any other proteins in stoichiometric amounts ( Fig. 1a ). In addition, affinity-purified PCSS complexes from meiotic and mitotic cells have identical compositions. Absence of Psy3, but not Shu2, leads to loss of Csm2 from the complex without affecting Shu1 (lanes 2 and 3 in Supplementary Fig.S1b and lanes 3 and 4 in Supplementary Fig. S1d ). In contrast, deletion of the CSM2 gene causes loss of Shu2 from the Shu1-complex in vivo (lane 5 of Supplementary Fig. S1b ). These observations suggest in vivo physical interactions between Psy3–Csm2, Psy3–Shu1, Shu1–Shu2 and Csm2–Shu2. 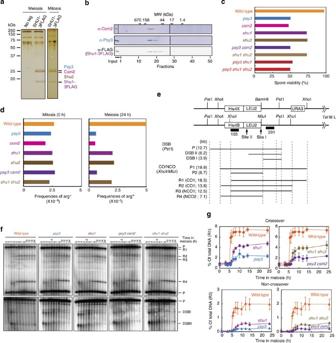Figure 1: PCSS forms a hetero-tetramer necessary for meiosis. (a) Affinity purification of Shu1-3FLAG. Fractions from mitotic and meiotic cells were analysed by silver staining. (b) Complex formation of the PCSS was examined by gel filtration of purified Shu1-3FLAG fractions. (c) Spore viability of variouspcssmutants (n=100). (d) Hetero-allelic recombination betweenarg4-bgland arg4-nspalleles was quantified by the ‘return-to-growth’ assay. The graphs show the frequencies of Arg+prototrophs at 0 (left) and 24 (right) hours after the induction of meiosis (n=2). (e) Schematic representation of theHIS4-LEU2recombination hotspot assay locus located onS. cerevisiaechromosome 3. DiagnosticXhoI (X) restriction-site polymorphisms and the position of the probe are shown. The size and composition of detected DNA species are shown below. Each line represents a DNA duplex. (f) Physical analysis of repair of meiotic double-strand breaks (lower panels) and the formation of crossovers and non-crossovers (upper panels) in meiotic recombination. (g) Quantification of crossovers (R1) and non-crossovers (R3) inf. An average of three independent time courses is shown with error-bars (s.d). Figure 1: PCSS forms a hetero-tetramer necessary for meiosis. ( a ) Affinity purification of Shu1-3FLAG. Fractions from mitotic and meiotic cells were analysed by silver staining. ( b ) Complex formation of the PCSS was examined by gel filtration of purified Shu1-3FLAG fractions. ( c ) Spore viability of various pcss mutants ( n =100). ( d ) Hetero-allelic recombination between arg4-bgl and arg4- nsp alleles was quantified by the ‘return-to-growth’ assay. The graphs show the frequencies of Arg + prototrophs at 0 (left) and 24 (right) hours after the induction of meiosis ( n =2). ( e ) Schematic representation of the HIS4-LEU2 recombination hotspot assay locus located on S. cerevisiae chromosome 3. Diagnostic Xho I (X) restriction-site polymorphisms and the position of the probe are shown. The size and composition of detected DNA species are shown below. Each line represents a DNA duplex. ( f ) Physical analysis of repair of meiotic double-strand breaks (lower panels) and the formation of crossovers and non-crossovers (upper panels) in meiotic recombination. ( g ) Quantification of crossovers (R1) and non-crossovers (R3) in f . An average of three independent time courses is shown with error-bars (s.d). Full size image The PCSS complex is required for meiotic recombination Previous genetic studies suggested a role for the PCSS proteins in the HR-dependent repair of replication forks [14] . In addition, the csm2 mutant was reported to have a defect in chromosome segregation during meiosis [12] , for which HR has an essential role. We performed a detailed characterization of the meiotic phenotypes of the four pcss mutants. Amounts of Csm2 and Psy3 proteins are constant during meiosis ( Supplementary Fig. S1e ). All four mutants decrease spore viability ( Fig. 1c ). The psy3 and csm2 mutants show a ~two-fold decrease in spore viability (50% and 47%, respectively, P -value <0.01, compared with 97% in wild-type) and spore viability of the psy3 csm2 double mutant is similar to that of each single mutant, indicating that Psy3 and Csm2 work together. In contrast, the shu1 and shu2 single mutants produce significantly more viable spores (73% and 74%, respectively; P -value <0.01 relative to psy3 and csm2 mutants), and viability of the shu1 shu2 double mutant (69%) suggests that Shu1 and Shu2 work together. Spore viability of a psy3 shu1 double mutant and a psy3 shu1 shu2 triple mutant implies that psy3 is epistatic to the shu1 and shu2 mutations. These data suggest that Psy3-Csm2 has a more fundamental role in the PCSS complex than does Shu1-Shu2. Analysis of recombination between arg4 hetero-alleles by a return-to-growth assay shows that all pcss mutants reduce the frequency of Arg + prototroph formation. psy3 and csm2 mutations decrease the frequency by 10-fold compared with wild-type, while shu1 and shu2 decrease Arg + prototrophs by only 2-fold ( Fig. 1d ). These data indicate that PCSS is required for efficient commitment to recombination in meiosis. The timing and efficiency of landmark events in meiosis were examined using synchronous meiotic time courses of various pcss single and double mutants. In psy3 , csm2 single, and psy3 csm2 and shu1 shu2 double mutants, the first meiotic division is delayed by 5 h compared with wild-type ( Supplementary Fig. S2a ). shu1 , shu2 single and shu1 shu2 double mutants show a 4-h delay. All of the mutants show a slight delay (≤1 h) in the completion of meiotic-S-phase ( Supplementary Fig. S2b ), consistent with the reported role of PCSS proteins in mitotic S-phase [10] , [14] . Physical monitoring of meiotic recombination intermediates was performed at the HIS4-LEU2 recombination hotspot [17] ( Fig. 1e ). psy3 and shu1 single mutants show normal appearance of DSBs relative to wild-type (lower panels of Fig. 1f ); however, the disappearance of DSBs is delayed by 2 and 1 h, respectively, indicating that pcss mutations delay the repair of meiotic DSBs. Consistently, recombination products, both crossovers and non-crossovers, form with similar delays and are greatly reduced relative to wild-type ( Fig. 1f , and also see Fig. 2 ). Crossover levels are reduced by 50% in shu1 strains and by 75% in psy3 relative to wild-type. Thus, PCSS proteins are required for efficient meiotic recombination and, in this respect, Psy3 is more important than Shu1. Consistent with our suggestion of Psy3–Csm2 and Shu1–Shu2 sub-complexes, recombination phenotypes of a shu1 shu2 double mutant are very similar to those of the shu1 single mutant and psy3 csm2 is similar to psy3 ( Fig 1f ). 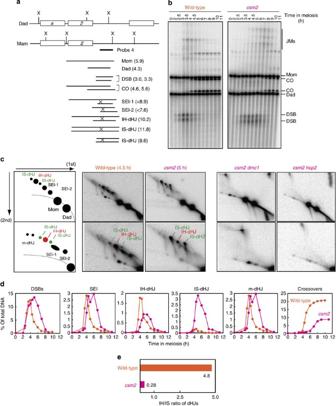Figure 2: PCSS promotes inter-homolog recombination during meiosis. (a) Schematic representation of theHIS4-LEU2recombination hotspot assay locus for 2D assay. (b) Southern blot images of one-dimensional (1D) gel analysis of meiotic recombination in wild-type andcsm2strains. Genomic DNA samples at each time point were digested withXhoI, separated on an agarose gel, and visualized by Southern blotting. (c) Southern images of two-dimensional (2D) gel analysis of JM intermediates, single-end invasions (SEIs) and double-Holliday junctions (dHJs). No JMs are detected incsm2 dmc1andcsm2 hop2strains (right-hand side panels), showing that strand-exchange in thecsm2mutant is completely dependent on Dmc1 and its accessory complex, Hop2(-Mnd1). (d) Temporal analysis of DSB, SEI, IH-dHJ, IS-dHJ, multi-chromatid JMs (m-JM), and crossovers are shown for wild-type (orange) andcsm2(magenta) strains Representative results are shown (n=3). (e) A ratio of IH-dHJ to IS-dHJ in wild-type andcsm2is shown. Figure 2: PCSS promotes inter-homolog recombination during meiosis. ( a ) Schematic representation of the HIS4-LEU2 recombination hotspot assay locus for 2D assay. ( b ) Southern blot images of one-dimensional (1D) gel analysis of meiotic recombination in wild-type and csm2 strains. Genomic DNA samples at each time point were digested with Xho I, separated on an agarose gel, and visualized by Southern blotting. ( c ) Southern images of two-dimensional (2D) gel analysis of JM intermediates, single-end invasions (SEIs) and double-Holliday junctions (dHJs). No JMs are detected in csm2 dmc1 and csm2 hop2 strains (right-hand side panels), showing that strand-exchange in the csm2 mutant is completely dependent on Dmc1 and its accessory complex, Hop2(-Mnd1). ( d ) Temporal analysis of DSB, SEI, IH-dHJ, IS-dHJ, multi-chromatid JMs (m-JM), and crossovers are shown for wild-type (orange) and csm2 (magenta) strains Representative results are shown ( n =3). ( e ) A ratio of IH-dHJ to IS-dHJ in wild-type and csm2 is shown. Full size image To understand why recombination products are reduced in pcss mutants, we also analysed joint molecule (JM) strand-exchange intermediates, single-end invasions [18] and double-Holiday junctions (dHJs) [19] at the HIS4–LEU2 recombination hotspot ( Fig. 2a ) by one and two-dimensional electrophoresis. The csm2 mutant shows delays in the formation and turnover of single-end invasions and dHJs compared with wild-type ( Fig. 2b–d ). Strikingly, most JMs are formed between sister-chromatids in csm2 cells ( Fig. 2c ). Although wild-type cells form inter-homologue dHJs (IH-dHJs) with a bias of 5:1 over inter-sister dHJs (IS-dHJs), csm2 mutants have reduced IH-dHJs and form up to 10-fold more IS-dHJs resulting in an inverted ratio of 0.28 ( Fig. 2e ). A similar loss of inter-homologue bias was previously demonstrated for rad51 mutants [20] . Indeed, like rad51 mutants, JM formation in the csm2 mutant is completely dependent on meiosis-specific RecA homologue, Dmc1 and its partner Hop2 ( Fig. 2c ) [21] , [22] . pcss mutants are defective in Rad51-assembly Although the recombination phenotypes of pcss mutants resemble those of rad51 null mutants, pcss cells produce 50–75% viable spores ( Fig. 1c ), whereas rad51 spores are dead [23] . To further understand the relationship between PCSS and Rad51, we monitored the chromosomal localization of Rad51 and Dmc1, by immunofluorescence microscopy [21] , [23] , [24] ( Fig. 3a ). In wild-type cells, a punctate pattern of immuno-staining foci is seen for both Rad51 and Dmc1 ( Fig. 3a ) [25] , [26] . Strikingly, all four pcss single mutants are defective in the formation of Rad51 foci. For example, the average number of Rad51 foci per nucleus in psy3 mutant cells is 6.7+/−5.7 ( n =41) foci at 4 h compared with 42+/−12 foci ( n =60) in wild-type. Low numbers of Rad51 foci were also observed in shu1 shu2 and psy3 csm2 double mutants (upper panels of Fig. 3b ). In addition, the psy3 and csm2 mutants significantly reduce the overall fraction of nuclei that contain any Rad51 foci, a phenotype that was not observed for the shu1 and shu2 mutants (lower panels of Fig. 3b ). These results show that the PCSS proteins are necessary for efficient assembly of Rad51 complexes on meiotic chromosomes. 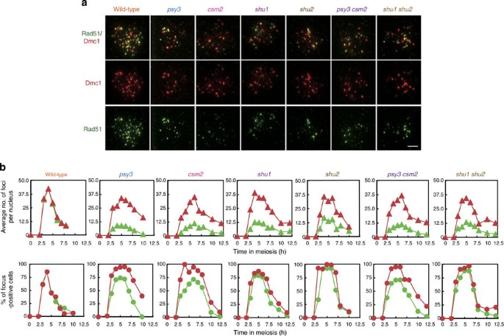Figure 3: PCSS promotes Rad51-assembly on meiotic chromosomes. (a) Immuno-staining analysis of Rad51 and Dmc1 foci on meiotic chromosome spreads. Green, Rad51; Red, Dmc1. Scale Bar, 2 μm. (b) Kinetic analysis of Rad51 and Dmc1 foci. Percents of focus-positive cells (bottom) and an average number of the focus per focus-positive nucleus (top) are shown at each time point. A focus-positive nucleus is defined as spreads with more than 5 foci. Representative results are shown (n=3). Figure 3: PCSS promotes Rad51-assembly on meiotic chromosomes. ( a ) Immuno-staining analysis of Rad51 and Dmc1 foci on meiotic chromosome spreads. Green, Rad51; Red, Dmc1. Scale Bar, 2 μm. ( b ) Kinetic analysis of Rad51 and Dmc1 foci. Percents of focus-positive cells (bottom) and an average number of the focus per focus-positive nucleus (top) are shown at each time point. A focus-positive nucleus is defined as spreads with more than 5 foci. Representative results are shown ( n =3). Full size image On the other hand, peak steady state numbers of Dmc1 foci are only slightly reduced in pcss mutants relative to wild-type (upper panels of Fig. 3b ). This observation is consistent with the fact that Rad51 facilitates the assembly of Dmc1 complexes [25] , [26] . Kinetic analysis shows that the disappearance of both Dmc1 and Rad51 foci is delayed in pcss mutant cells ( Fig. 3b ). The psy3 and csm2 mutants cause a greater delay than shu1 and shu2 mutants, consistent with our analysis of the timing of recombination above. Taken together, our cytological analysis indicates that assembly of Rad51 and Dmc1 complexes is uncoupled in pcss mutants: although Dmc1 foci form almost normally, Rad51 focus formation is severely defective. Recently, the budding yeast Rad51-paralogues, Rad55-Rad57, were shown to stabilize Rad51-filaments by antagonizing Srs2, which translocates along ssDNA and displaces Rad51 (ref. 6 ). A similar role for the PCSS proteins in mitotic recombination and DSB repair has been suggested [12] , [14] , [15] . To test this proposal, we asked whether deletion of the SRS2 gene is able to suppress the Rad51-assembly defect of the psy3 mutant. Deletion of the SRS2 gene alone slightly reduces the number of Rad51 immuno-staining foci ( Fig. 4a ). However, srs2 psy3 double mutants have the same number of Rad51 foci as seen in the psy3- single mutant ( Fig. 4b ; P -value=0.56; Mann–Whitney’s U -test), implying that Srs2 is not responsible for the defective Rad51 assembly seen in pcss mutants. This analysis was extended by physical analysis of meiotic recombination ( Fig. 4d ), which shows that srs2 mutation does not suppress the recombination defects of pcss mutant cells (see also Fig. 1f ). Consistent with this analysis, srs2 mutation does not suppress delay in the delayed meiotic entry of the psy3 mutant cells ( Fig. 4c ). Thus, the PCSS complex does not appear to promote Rad51 function during meiosis by antagonizing Srs2. However, we can not rule out the possibility that the PCSS complex may have dual functions: antagonizing Srs2 in mitotic cycling cells and promoting Rad51-assembly in meiosis. 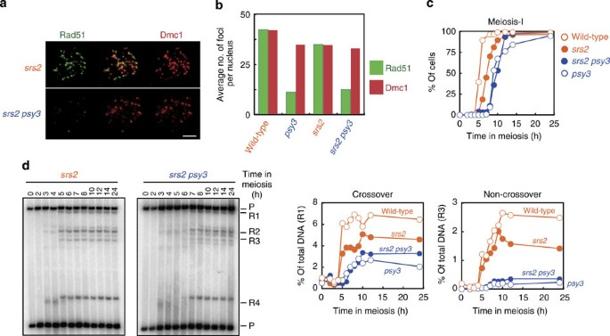Figure 4: Thesrs2mutation does not suppresspsy3defects in meiosis. (a) Representative meiotic nuclei immuno-stained for Rad51 (green) and Dmc1 (red) in thesrs2andsrs2 psy3mutant backgrounds. (b) Average number of Rad51 (green) or Dmc1 (red) foci per focus-positive nucleus in wild-type (4 h),psy3(5 h),srs2(5 h) andsrs2 psy3(5 h) strains. A focus-positive nucleus is defined as having >5 foci. Representative results are shown (n=3). Statistical differences are shown in main text. (c) Timing of meiotic division I in wild-type and various mutant cells was measured by DAPI staining. (d) Southern blot images of 1D gels analysing crossovers and non-crossovers (left). Quantification of meiotic divisions, and crossover (R1) and non-crossover (R3) levels determined by Southern blot analysis. Representative results are shown (n=3). Wild-type (open orange circles),psy3(open blue circles),srs2(closed orange circles) andsrs2 psy3(closed blue circles). Figure 4: The srs2 mutation does not suppress psy3 defects in meiosis. ( a ) Representative meiotic nuclei immuno-stained for Rad51 (green) and Dmc1 (red) in the srs2 and srs2 psy3 mutant backgrounds. ( b ) Average number of Rad51 (green) or Dmc1 (red) foci per focus-positive nucleus in wild-type (4 h), psy3 (5 h), srs2 (5 h) and srs2 psy3 (5 h) strains. A focus-positive nucleus is defined as having >5 foci. Representative results are shown ( n =3). Statistical differences are shown in main text. ( c ) Timing of meiotic division I in wild-type and various mutant cells was measured by DAPI staining. ( d ) Southern blot images of 1D gels analysing crossovers and non-crossovers (left). Quantification of meiotic divisions, and crossover (R1) and non-crossover (R3) levels determined by Southern blot analysis. Representative results are shown ( n =3). Wild-type (open orange circles), psy3 (open blue circles), srs2 (closed orange circles) and srs2 psy3 (closed blue circles). Full size image PCSS binds to recombination intermediates We tried to localize PCSS proteins on meiotic chromosome spreads by immuno-staining, but failed to detect any specific signals. Instead, we examined the association of PCSS proteins with recombination hotspots by chromatin immuno-precipitation (ChIP). Using the PSY3-3FLAG strain, we observe that Psy3 specifically binds the HIS4–LEU2 recombination hotspot, but not to a control locus, SMC1 ( Fig. 5a ). Mock analysis of an untagged strain shows that the ChIP signals are specific to Psy3-3FLAG ( Fig. 5a ). Robust binding of Psy3 to HIS4-LEU2 is seen only at 4 h, when Rad51 also binds to the hotspot ( Fig. 5c ). A similar ChIP-binding profile is seen for the Shu1-3FLAG strain ( Fig. 5d ). Binding of Psy3-3FLAG to the recombination hotspot is dependent of DSB formation, as shown by ChIP analysis of a spo11-Y135F strain, which is defective for DSB formation ( Fig. 5b ). Interestingly, absence of Rad51 does not abolish hotspot binding of Psy3 and Shu1, but delays their dissociation ( Fig. 5b ). Elimination of the Rad51-paralogues, Rad55(-Rad57), abolishes Rad51-binding ( Fig. 5c ), but does not affect the association of Psy3 with the HIS4-LEU2 hotspot ( Fig. 5b ). The delayed dissociation of Psy3 in the rad51 and rad55 mutants is consistent with the delayed repair of meiotic DSBs in these mutants. Consistent with our cytological analysis, above, psy3 mutation completely abolishes the recruitment of Rad51 to the recombination hotspot, ( Fig. 5c ) but does not affect the binding of Dmc1 ( Fig. 5e ). ChIP signals for Shu1 are also diminished in psy3 mutants ( Fig. 5d ). In contrast, in the shu1 mutant, which also abolishes Rad51 binding, Psy3 can still associate with the recombination hotspot, with ChIP signals at ~60% of those detected in wild-type ( Fig. 5b ). These data indicate that the PCSS complex promotes assembly of Rad51 at recombination sites and show that PCSS binds recombination intermediates in a manner that is independent of both Rad51 and the Rad55–Rad57 complex. 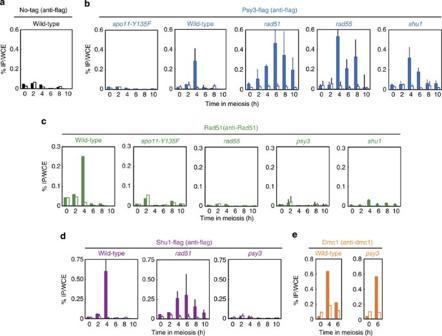Figure 5: PCSS promotes Rad51-assembly on recombination intermediates. Chromatin-immunopreciptation (ChIP) analyses of control (a, black), Psy3-3FLAG (b, blue), Rad51 (c, green), Shu1-3FLAG (d, purple), and Dmc1 (e, orange) were carried out in different strains. Binding efficiencies (% of immuno-precipitated to whole-cell lysates) of each protein to a region in theHIS4-LEU2recombination hotspot (closed bars) and a control region of internal region of theSMC1ORF (open bars) are shown. In some experiments, s.d. (n=3) is shown. Figure 5: PCSS promotes Rad51-assembly on recombination intermediates. Chromatin-immunopreciptation (ChIP) analyses of control ( a , black), Psy3-3FLAG ( b , blue), Rad51 ( c , green), Shu1-3FLAG ( d , purple), and Dmc1 ( e , orange) were carried out in different strains. Binding efficiencies (% of immuno-precipitated to whole-cell lysates) of each protein to a region in the HIS4-LEU2 recombination hotspot (closed bars) and a control region of internal region of the SMC1 ORF (open bars) are shown. In some experiments, s.d. ( n =3) is shown. Full size image Psy3-Csm2 is structurally similar to the Rad51 dimer Informed by our genetic analysis, we found that Psy3-Csm2 and Shu1-Shu2 combinations expressed well in E. coli and were readily purified as stable sub-complexes ( Fig. 6a ). Gel filtration shows that each sub-complex elutes at the size expected for hetero-dimers ( Fig. 6b ). Electrophoresis mobility shift (EMS) analysis indicates that Psy3-Csm2, but not Shu1-Shu2, can bind to both ϕX174 ss- and ds-DNAs in a concentration-dependent manner ( Fig. 6c ), indicating non-specific DNA binding. DNA binding by Psy3-Csm2 occurs independently of a nucleotide such as ATP (see Supplementary Fig. S3 ). To date, our attempts to detect direct protein–protein interaction between Rad51 and Psy3-Csm2, both in vivo and in vitro using purified proteins, have failed. 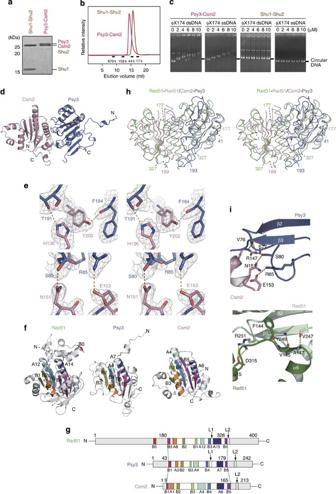Figure 6: Crystal structure of Psy3-Csm2 dimer. (a) Each 1 μg of purified fractions of Psy3-Csm2 and Shu1-Shu2 are analysed on SDS–PAGE gel and visualized with the Coomassie staining. (b) A profile of gel filtration using Superdex200 of Psy3-Csm2 (magenta) and Shu1-Shu2 (brown) are shown with size markers. (c) The binding of either Psy3-Csm2 or Shu1-Shu2 to ss- or dsDNAs (ϕX174 DNA, 135 μM) was studied by EMS assay. Protein–DNA complexes were resolved in a 0.8% agarose gel and were visualized with EtBr-staining. (d) A crystal structure of Psy3-Csm2 dimer is shown in a ribbon-presentation. Csm2, pink; Psy3, blue. (e) A stereo view of an interface between Psy3 (blue) and Csm2 (pink) is shown. Maps (2Fo-Fc) are shown at 1.5σ contour levels.(f)Structural comparison among Rad51 protomer (left), Psy3 (middle) and Csm2 (right). Homologous α-helixes and β-sheets are shown in colours. (g) Schematic comparison of domains among Rad51, Psy3 and Csm2. Two loops, L1 and L2, are DNA binding regions of Rad51 and homologous loops to L1 and L2 are shown for Psy3 and Csm2. (h) Comparison of Psy3-Csm2 with Rad51 dimer. Csm2, pink; Psy3, blue. Rad51 dimer (1SZP) is shown in green (right monomer, chain B in 1SZP) and light green (left monomer, chain C in 1SZP). Super-imposition of Rad51 with Psy3-Csm2 dimer is indicated as a stereo view. Psy3-Csm2 is simply superimposed with Rad51 dimer using COOT. (i) The interface between Psy3 and Csm2 (top) is compared with that between Rad51 (green) and Rad51 (light green) protomers (bottom). Figure 6: Crystal structure of Psy3-Csm2 dimer. ( a ) Each 1 μg of purified fractions of Psy3-Csm2 and Shu1-Shu2 are analysed on SDS–PAGE gel and visualized with the Coomassie staining. ( b ) A profile of gel filtration using Superdex200 of Psy3-Csm2 (magenta) and Shu1-Shu2 (brown) are shown with size markers. ( c ) The binding of either Psy3-Csm2 or Shu1-Shu2 to ss- or dsDNAs (ϕX174 DNA, 135 μM) was studied by EMS assay. Protein–DNA complexes were resolved in a 0.8% agarose gel and were visualized with EtBr-staining. ( d ) A crystal structure of Psy3-Csm2 dimer is shown in a ribbon-presentation. Csm2, pink; Psy3, blue. ( e ) A stereo view of an interface between Psy3 (blue) and Csm2 (pink) is shown. Maps (2Fo-Fc) are shown at 1.5σ contour levels. (f) Structural comparison among Rad51 protomer (left), Psy3 (middle) and Csm2 (right). Homologous α-helixes and β-sheets are shown in colours. ( g ) Schematic comparison of domains among Rad51, Psy3 and Csm2. Two loops, L1 and L2, are DNA binding regions of Rad51 and homologous loops to L1 and L2 are shown for Psy3 and Csm2. ( h ) Comparison of Psy3-Csm2 with Rad51 dimer. Csm2, pink; Psy3, blue. Rad51 dimer (1SZP) is shown in green (right monomer, chain B in 1SZP) and light green (left monomer, chain C in 1SZP). Super-imposition of Rad51 with Psy3-Csm2 dimer is indicated as a stereo view. Psy3-Csm2 is simply superimposed with Rad51 dimer using COOT. ( i ) The interface between Psy3 and Csm2 (top) is compared with that between Rad51 (green) and Rad51 (light green) protomers (bottom). Full size image We were able to crystallize purified Psy3-Csm2 and solve its structure with a resolution of 2.0 Å ( Supplementary Table S1 ). The structure confirms that Psy3-Csm2 is indeed a stable hetero-dimer ( Fig. 6d ). Psy3 and Csm2 contain an α/β barrel structure with an extensive hydrogen-bonded interface between Csm2 and Psy3 ( Fig. 6e ). Homology search reveals that Psy3 and Csm2 structures are highly homologous with each other despite their lack of amino-acid sequence homology ( Fig. 6f ; Supplementary Fig. S5a ). Importantly, Psy3 and Csm2 are structurally similar to Rad51 [1] , [27] and, thus, to bacterial RecA and archeal RadA ( Fig. 6f ; Supplementary Fig. S5a ). At the amino-acid sequence level, neither Psy3 nor Csm2 show significant homology to Rad51/RecA, or other Rad51 paralogues, all of which contain Walker A and B-type motifs for nucleotide binding ( Supplementary Figs S4,S6 ). Indeed, a typical nucleotide-binding fold is not present in these proteins, although the overall folds of Csm2 and Psy3 are quite similar to the Rad51/RecA family. These structural features are consistent with our observations that the binding of Psy3-Csm2 to DNA occurs independently of nucleotide cofactor whereas that of Rad51 requires ATP or a related analogue ( Supplementary Fig. S3 ). Similar structures for Psy3-Csm2 have been recently reported by two-independent groups [28] , [29] . The Psy3-Csm2 dimer shares striking structural homology to the Rad51 dimer [1] ( Fig. 6h and Supplementary Fig. S5b ). Rice et al . [1] proposed that the Rad51 dimer is the fundamental unit of the Rad51 nucleoprotein filament. In the Rad51 dimer, each protomer of Rad51 interacts in a way that is modulated by ATP. In the filament, dimers use different interfaces for interaction with adjacent Rad51 protomers [1] , [27] . In the dimeric structure, an interface between Psy3 and Csm2 is very similar to that of a Rad51 monomer–monomer ( Fig. 6i ). Psy3 and Csm2 are homologous to a core domain (180–326) of Rad51 ( Fig. 6g ). In Rad51, this core domain contains ATP- and DNA-binding domains (L1 and L2 loops) as well as an interface with an adjacent Rad51 protomer in the filament ( Supplementary Fig. S6 ). Rad51 bears N- and C-terminus extensions that are not present in Psy3 and Csm2. In the N-terminus of Rad51, there is a second interface for the Rad51 dimer as well as a dsDNA-binding domain ( Supplementary Fig. S6 ). Using model building, we replaced a single Rad51 dimer in the Rad51 filament with Psy3-Csm2 and observed a good structural fit ( Fig. 7a ). The Rad51 filament has a defined polarity although the direction of Rad51 polymerization has not been determined definitively. Thus, theoretically, the Psy3-Csm2 dimer could be placed at either the 5′- or the 3′-end of the Rad51 filament, or even within the filament. However, because of difficulty in structural fitting between Rad51 and Psy3, we favour placement of the Psy3-Csm2 dimer at the 5′-end of the Rad51 filament, with Csm2 facing Rad51. Our modelling is supported by the recent SAXS analysis of the PCSS complex, which shows rough location of Shu1-Shu2 in respect of Psy3-Csm2 (ref. 28 ). Indeed, Shu1-Shu2 is likely to be positioned on the side of Psy3 ( Fig. 7b ), which may confer steric hindrance for the accessibility of other protein(s); for example, Rad51 to Psy3. 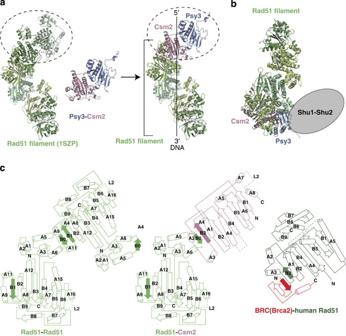Figure 7: A model of Psy3-Csm2 to promote Rad51-filament formation. (a) A top Rad51 dimer in Rad51 filament (1SZP) with 6 Rad51 protomers (green; left) was replaced with Psy3-Csm2 (blue-pink; middle) after the structural fit of the Psy3-Csm2 to the Rad51 dimer (right). (b) The position of a mass with Shu1-Shu2 dimer (grey oval) in Psy3-Csm2-Shu1-Shu2 (Sheet al, 2012) is placed on the putative Rad51 filament with Psy3-Csm2. Compared with the model ina, the structure is rotated by 180°. (c) An interface between yeast Rad51 and yeast Rad51 (green; left), human Rad51 and a BRC repeat of human Brca2 (right) is shown in topographic representation. A putative interface between Rad51 (green) and Csm2 (pink) is presented in the middle. Rad51-Rad51 and human Rad51-BRC is from 1SPZ and 1N0W, respectively. Figure 7: A model of Psy3-Csm2 to promote Rad51-filament formation. ( a ) A top Rad51 dimer in Rad51 filament (1SZP) with 6 Rad51 protomers (green; left) was replaced with Psy3-Csm2 (blue-pink; middle) after the structural fit of the Psy3-Csm2 to the Rad51 dimer (right). ( b ) The position of a mass with Shu1-Shu2 dimer (grey oval) in Psy3-Csm2-Shu1-Shu2 (She et al , 2012) is placed on the putative Rad51 filament with Psy3-Csm2. Compared with the model in a , the structure is rotated by 180°. ( c ) An interface between yeast Rad51 and yeast Rad51 (green; left), human Rad51 and a BRC repeat of human Brca2 (right) is shown in topographic representation. A putative interface between Rad51 (green) and Csm2 (pink) is presented in the middle. Rad51-Rad51 and human Rad51-BRC is from 1SPZ and 1N0W, respectively. Full size image In the filament, an N-terminal β-sheet (β-sheet 0; B0) of Rad51 aligns in an anti-parallel configuration with a β-sheet (β-sheet 1; B1) of the core region of the adjacent Rad51 protomer [1] , [27] ( Fig. 7c , left). Csm2 may provide a β-sheet, which mimics β-sheet 1 of Rad51 that interfaces with the β-sheet 0 domain of Rad51 ( Fig. 7c , middle). This modelling suggests that Psy3-Csm2, and by inference the PCSS complex, may interact with only one end of the Rad51 filament. It is interesting to note the inferred site of interaction between Csm2 and Rad51 is completely opposite to the Rad51 interface with Brca2 (Breast cancer responsible gene 2; Fig. 7c , right). Like the Psy3-Csm2 dimer, Brca2 is known to stabilize the Rad51-filament, possibly by binding to one end [27] , [30] . Psy3-Csm2 stabilizes Rad51 filaments in vitro The above structural model combined with various results presented here suggests that the Psy3-Csm2 dimer may stabilize a Rad51 filament by binding the end. However, it is technically difficult to analyse the stability of the Rad51 filament, for example, extension of Rad51 filament stabilizes itself. If our model is true ( Fig. 7 ), the Psy3-Csm2 dimer stabilizes only one Rad51 protomer located at the filament end. Therefore, we need to develop a sensitive assay to detect the effect of Psy3-Csm2 on the stability of Rad51 filament. We first examined the formation of a ternary complex of Rad51 and Psy3-Csm2 on ssDNAs by the EMS assay using a short oligo-ssDNA ( Fig. 8a ). Rad51 forms a stable complex with a 60-mer ssDNA in the presence of ATP, but not in the presence of ADP or in the absence of nucleotide cofactor, showing that ATP stabilizes the Rad51–ssDNA complex, and thus the Rad51 filament ( Fig. 8a ), consistent with previous reports [31] . Under the same conditions, Psy3–Csm2–DNA complexes are trapped in the well of the gel, suggesting the formation of aggregates with the DNA. Co-incubation of oligo-DNA with Rad51 and Psy3-Csm2 generates a novel species on the gel, whose appearance depends upon the concentration of each protein ( Fig. 8a ). This indicates formation of a co-complex, which contains both Rad51 and Psy3-Csm2. Addition of either anti-Rad51 or anti-Psy3 antibody produced a super-shifted species, indicating that the complex contains both Rad51 and Psy3 ( Fig. 8b ). 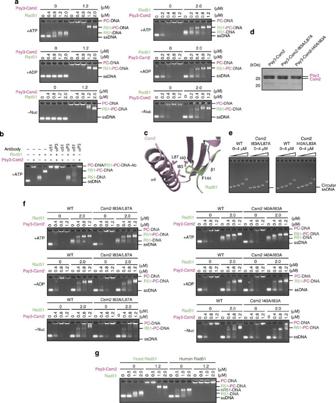Figure 8: Psy3-Csm2 dimer binds DNAs and stabilizes Rad51–DNA complex. (a) Co-complex formation of Rad51 and Psy3-Csm2 on DNA was analysed in EMS assay. Different concentrations of Rad51 and Psy3-Csm2 are incubated with a FITC-labelled 60 mer ssDNA (6 μM in nucleotide) in the presence of 1 mM ATP (top), 1 mM ADP (middle) and in the absence of any nucleotides (bottom). The complexes were resolved in a 0.8% agarose containing 1 mM MgCl2. Protein–DNA complexes were analysed with an image analyser. PC, Psy3-Csm2; R51; Rad51. (b) Antibodies against Rad51 and Psy3 were added to check the presence of each protein in the complex. The antibodies were added after the complex formation. (c) A putative interface of Rad51 (green) and Csm2 (pink) is shown with possible amino acids of Csm2 responsible to Rad51-binding. (d). Purification of Psy3-Csm2-I83A/L87A and Psy3-Csm2-I40A/I83A. One micro-gram of purified complexes was analysed on SDS–PAGE. (e) EMS analysis of DNA binding of Psy3-Csm2-I83A/L87A and Psy3-Csm2-I40A/I83A. (f) Effects of Psy3-Csm2-I83A/L87A and Psy3-Csm2-I40A/I83A proteins on Rad51-filament stabilization. The analysis was carried out as shown (a). (g) Different concentrations of yeast and human Rad51 were incubated with the oligo-DNA and ATP in the absence or the presence of Psy3-Csm2. Products were analysed on an agarose gel. Yeast Rad51, green: human Rad51, deep green. Figure 8: Psy3-Csm2 dimer binds DNAs and stabilizes Rad51–DNA complex. ( a ) Co-complex formation of Rad51 and Psy3-Csm2 on DNA was analysed in EMS assay. Different concentrations of Rad51 and Psy3-Csm2 are incubated with a FITC-labelled 60 mer ssDNA (6 μM in nucleotide) in the presence of 1 mM ATP (top), 1 mM ADP (middle) and in the absence of any nucleotides (bottom). The complexes were resolved in a 0.8% agarose containing 1 mM MgCl 2 . Protein–DNA complexes were analysed with an image analyser. PC, Psy3-Csm2; R51; Rad51. ( b ) Antibodies against Rad51 and Psy3 were added to check the presence of each protein in the complex. The antibodies were added after the complex formation. ( c ) A putative interface of Rad51 (green) and Csm2 (pink) is shown with possible amino acids of Csm2 responsible to Rad51-binding. ( d ). Purification of Psy3-Csm2-I83A/L87A and Psy3-Csm2-I40A/I83A. One micro-gram of purified complexes was analysed on SDS–PAGE. ( e ) EMS analysis of DNA binding of Psy3-Csm2-I83A/L87A and Psy3-Csm2-I40A/I83A. ( f ) Effects of Psy3-Csm2-I83A/L87A and Psy3-Csm2-I40A/I83A proteins on Rad51-filament stabilization. The analysis was carried out as shown ( a ). ( g ) Different concentrations of yeast and human Rad51 were incubated with the oligo-DNA and ATP in the absence or the presence of Psy3-Csm2. Products were analysed on an agarose gel. Yeast Rad51, green: human Rad51, deep green. Full size image The stabilization effect of Psy3-Csm2 on the Rad51–DNA complex is seen only when the filament becomes unstable ( Fig. 8a ). As described previously, the EMS assay shows that Rad51-filaments are more stable in the presence of ATP than in the presence of ADP and in the absence of any nucleotides; Rad51 can not form stable ssDNA complexes. However, the addition of Psy3-Csm2 produced a co-complex with Rad51 even in the presence of ADP or in the absence of nucleotide (‘+ADP’ or ‘−nuc’, Fig. 8a ). In addition, the ternary complex formed in the presence of ATP is more resistant to salt compared with the Rad51–ssDNA complex alone ( Supplementary Fig. S7a ). These data suggest that Psy3-Csm2 stabilizes the Rad51–ssDNA complex by forming a co-complex on DNA. Structural prediction suggests that the Csm2 of the Psy3-Csm2 dimer provides an interface with a Rad51 protomer ( Fig. 7c , 8c ) and that hydrophobic amino acids of I40, I83 and L87 of Csm2 may have a role in the interaction with Rad51. Thus, we constructed two mutant derivatives of Csm2, which have substitutions of amino acids at this putative Rad51 interface ( Fig. 8c ). Both Csm2-I83A/L87A and Csm2-I40A/I83A mutant proteins form a stable dimer with Psy3 and bind to ssDNA with similar binding affinity to the wild-type dimer ( Fig. 8d and Supplementary Fig. S7b ). Importantly, both Psy3-Csm2-I83A/L87A and Psy3-Csm2-I40A/I83A show reduced formation of a stable complex with Rad51 in the presence of ADP and in the absence of nucleotide cofactors relative to wild-type Psy3-Csm2 ( Fig. 8f ). These data suggest that Psy3-Csm2-I83A/L87A and Psy3-Csm2-I40A/I83A are partially defective in co-complex formation with Rad51 and Rad51-filament stabilization in vitro . We speculate that these residues are important, but not essential for the binding of Csm2 to Rad51 and other residues in this region (or other regions) may contribute to the binding of (Psy3-)Csm2 to Rad51. Alternatively, we may introduce hydrophilic substitutions on these residues to see a drastic effect. To support our inference of a specific functional interaction between Rad51 and Psy3-Csm2, we replaced yeast Rad51 with human Rad51 and assayed complex formation ( Fig. 8g ). In stark contrast to yeast Rad51, human Rad51 can not form a co-complex with yeast Psy3-Csm2. Rather Psy3-Csm2 competes with human Rad51 for DNA binding under these conditions. Our in vivo results suggest that the PCSS complex promotes the assembly of Rad51 onto RPA-coated ssDNAs (for example, Fig. 3 ). However, we did not include RPA in our EMS assay to reduce the complexity of the reaction. This might be an alternative reason why mutant Psy3–Csm2 complexes show a weak defect in Rad51-filament stabilization. Further experiments will be necessary to understand the precise mechanism of how the PCSS assists Rad51-assembly. Some components of the PCSS complex are evolutionally conserved in a variety of organisms including human [32] , [33] ( Supplementary Fig. S6a,6b ). Our structural analysis suggests that Psy3 and Csm2 are structural homologues of Rdl1 and Rlp1 in fission yeast [33] and to SWSAP1 in human [32] . Although Rdl1 and Rlp1 are not likely to be ATP-binding proteins, SWSAP1 is a Rad51 paralogue with an ATP-binding motif [32] ( Supplementary Fig. S6 ). Our studies also suggest that the PCSS and its paralogue (Rdl1-Rlp1) are unique in the use of an ATP-binding/hydrolysis independent activity for their mediator function when compared with other from other Rad51 paralogues (Rad51B etc). We have described a new Rad51-mediator in budding yeast, called PCSS. This hetero-tetramer promotes the assembly of functional Rad51 complexes during meiosis. PCSS is divided into two sub-complexes, Shu1-Shu2 and the DNA-binding core, Psy3-Csm2. Our in vivo and in vitro studies suggest that Psy3-Csm2 is a core sub-complex with Shu1-Shu2 as an accessory factor. Importantly, in vitro , Psy3-Csm2 can stabilize Rad51–DNA complexes independently of nucleotide cofactor. The crystal structure of Psy3-Csm2 reveals structural homology to the Rad51 dimer. Together, these studies reveal PCSS as a novel mediator of Rad51 nucleoprotein filament assembly, possibly by binding the 5′-end of the filament. The mechanism of PCSS action as a Rad51 mediator is distinct from that of other characterized mediators, such as Rad52, Rad55-Rad57 and Brca2 (refs 5 , 6 , 30 ), and suggest a paradigm for the mechanism of other Rad51 paralogues. In addition to a role of the PCSS complex in meiotic recombination, the complex also functions in Rad51/54-dependent post-replicative repair during S-phase [34] . The results described here suggest that the PCSS may facilitate the assembly of Rad51 filaments into unreplicated gaps behind replication forks that have bypassed DNA damage, or on a ‘Holliday junction-like-foot’ intermediate, formed by regression of the fork. Alternatively, the PCSS tetramer might have a non-mediator role during repair. Further studies are necessary to evaluate the function of the PCSS complex in replication fork repair during S-phase. In this respect, it is important to note that mammalian Brca2 and Rad51 have a role in the protection of ssDNA from degradation in S-phase cells containing DNA damage [35] , [36] . Given that budding yeast lacks a Brca2 homologue, it is possible that the PCSS has a similar role in the protection of replication forks. Previous genetic studies suggested that one role of PCSS is to antagonize the Srs2 helicase [15] , [29] . Our analysis of meiotic phenotypes of srs2 mutants argues against this idea ( Fig. 4 ). However, it remains possible that the PCSS complex has dual functions; antagonizing Srs2 in mitotically cycling cells and promoting Rad51-assembly during meiosis. Interestingly, another helicase, Mph1, belongs to the same epistasis group as the PCSS genes [16] . Further studies are necessary to evaluate the relationship between PCSS and Mph1. Yeast strains and yeast methods All yeast strains used in this paper are isogenic derivatives of SK1 and listed in Supplementary Table S2 . Media and culture conditions regarding meiosis were described [37] . DAPI staining and FACS analysis for DNA contents were also described previously [37] . For tetrad dissection, >100 tetrads were dissected. For return-to-growth experiment at the arg4 locus, meiotic cells taken from 0 and 12 h of meiosis were diluted in water and plated on SD-ARG and YPAD plates. The recombination frequency was calculated by counting the number of colonies on each plate. Cytological analysis and antibodies Immuno-staining was conducted as described [26] . Briefly, chromosome spreads were prepared from meiotic yeast cells and stained by primary and secondary antibodies [25] . Stained samples were observed using an epi-fluorescent microscope (AxioPlan; Zeiss with a × 100 objective (NA1.4). Images were captured by CCD camera (Retiga; Qimaging) at a room temperature, then processed using IP lab (Sillicon) software. Psuedo-coloring was performed using Photoshop (Adobe) software. At each time point, >50 spreads were analysed for focus-counting [25] . The primary antibody against Rad51 (Guinea Pig) and Dmc1 (Rabbit) was diluted at 1/500. The second antibodies conjugated with Alexa-fluor-488 (Goat) and −594 (Goat) IgG specific for primary antibodies (Invitrogen) were used at a 1/2000 dilution. Western and Southern Blotting Western blotting was performed for cell lysates extracted by the TCA method. After washing cell precipitates twice with 20% TCA, cells were roughly disrupted by bead-beater (Yasui Kikai Co Ltd, Japan). Protein precipitations recovered by centrifuge were suspended in a SDS–PAGE sample buffer and then boiled at 95 °C for 2 min. Anti-Csm2 and anti-Psy3 antibodies were raised against His-tagged proteins purified from E. coli . Southern blotting analysis was performed with the same procedure as described [38] . Genomic DNAs were digested with both Mlu I and Xho I (for crossover/non-crossover) and Pst I (for meiotic DSB, lower panels). Probes for Southern blotting were ‘Probe 155’ for crossover/non-crossover and ‘Probe 291’ for DSB detection as described [38] , [39] . Image Gauge software (Fuji film Co. Ltd., Japan) was used for quantification for bands of R1, R3 and DSB-I. Two-dimensional gel analysis for JMs was carried out as described [18] . Chromatin immuno-precipitation Cells were fixed with 2% of formaldehyde. Protein lysates were carried out as described above. Magnetic beads covered with anti-FLAG (M2, Sigma) or anti-Rad51 were incubated with the lysates. After incubation for overnight, the beads were recovered and washed extensively. DNAs were recovered with phenol/chroloform extraction and further purified with ethanol precipitation. In all, 1/10 of purified DNAs were subject to real-PCR reaction (BioRad iCycler) with Syber-Green as a dye. Two sets of paired primers were used for the assay. Primers for the HIS4-LEU2 and SMC1 loci were described [37] : HIS4-LEU2 for 5′-GACACCAGAGTTCAAATTCCAACGAG-3′ and 5′-CCAGCAGTTATTTATACTTGCAGCATC-3′; SMC1 for 5′-GGTGTGCGGAGTAATCATTTGAGG-3′ and 5′-TTATAGGAGACAGTTTTTCCATCAA-3′. Immuno-affinity purification Yeast cell lysates (from 500 ml culture) were prepared by the glass-bead disruption method [37] . The lysates were incubated with magnetic beads (Dynal M260, GE Health-care) coated with anti-FLAG antibodies antibody for 12 h and washed extensively. Bound proteins were eluted by the addition of 0.1 mg ml −1 of FLAG peptide. Protein expression and purification HIS 6 -PSY3 and CSM2 open reading frames are placed under the control of T7 promoter of an expression vector, pET28a. The vector, pMT, was introduced into E. coli , BL21(DE3) codon plus. Proteins were induced in cells cultured at 18 °C by the addition of IPTG for 16 h. Cells were disrupted by sonication and cell lystaes were applied to His-trap (GE Health-Care) for purification of the His-tagged proteins. After elution by a gradient of 40–250 mM imidazole, fractions containing His 6 -Psy3-Csm2 were incubated at room temperature with 400 μg protein per 1 unit of thrombin (GE Health-Care) for 16 h. Subsequently, fractions were subject to the following chromatographic fractionations; Psy3-Csm2; MonoQ. Hi-Trap Heparin; Shu1-Shu2; Hi-Trap, Heparin, MonoQ column. The resultant fractions were concentrated by ultrafiltration (Amicon-Ultra MWCO 30 k) and dialyzed with 25 mM HEPES pH7.0, 0.2 M KCl, 50% Glycerol, 1 mM EDTA, 1 mM DTT. From 20 g of E. coli cells, 10 mg of Psy3-Csm2 was obtained. Expression of Shu1-Shu2 hetero-dimer and its purification was essentially similar to those of Psy3-Csm2. Psy3-Csm2 containing L -Seleno-methionine (S-Met) was induced in E. coli cells with culture in S-Met minimum media supplemented with 25 mg ml −1 of S-Met. His 6 -Rad51 was overexpressed in BL21 (DE3) with pLysS. E. coli cell lysate was subject to the following steps; poly-ethylene-imin P precipitation followed by 0.5 M NaCl buffer washing and elution with 1.0 M NaCl buffer; (NH 4 ) 2 SO 4 precipitation; His-trap; thrombin treatment; MonoQ; Hi-trap Heparin. DNA binding 6 μM (in nucleotide) of a 60-mer oligo-nucleotide (5′-TGGGTGAACCTGCAGGTGGGCAAAGATGTCCTAGCAATCCATTGTCTATGACGTCAAGCT-3′) labelled with FITC at 5′-end were incubated with various concentrations of proteins in a 10 μl of buffer (20 mM Tris-HCl [7.5], 5 mM MgCl 2 , 50 μg ml-1 BSA, 1 mM ATP or ADP). After incubation for 10 min at 30 °C, and the applied into a 0.8% of agarose gel. Electrophoresis was carried out in 0.5X TAE buffer supplemented with 1 mM MgCl 2 for 30 min. DNA was visualized in an image analyser, LAS1,000 or LAS4,000 (Fuji, Co. Ltd). In the case of ϕX174 (135 μM for base-pair or nucleotide) as a substrate, after the electrophoresis in the 1X TAE buffer for 2 h, DNAs were visualized by staining with ethidium bromide. Mutant construction and purification Csm2-I83A/L87A and Csm2-I40A/I83A mutant genes were constructed by standard site-directed mutagenesis using the PCR. The mutant Csm2 proteins were co-expressed with Psy3. Psy3-Csm2 mutant complexes were purified to near homogeneity using the similar purification procedure for wild-type Psy3–Csm2 complex as described above. Crystallization and structure determination Crystallization of the Psy3-Csm2 and its Se-Met-containing derivative was performed as described. Purified Psy3-Csm2 dimer was subject to dialysis with 25 mM HEPES (pH7.5), 0.25 M NaCl, 10% Glycerol, 1 mM DTT for overnight. Dialysate was concentrated to 5 mg ml −1 using ultrafiltration (Amicon-Ultra MWCO 30 k). Crystals of native and Se-Met Psy3-Csm2 dimer were grown by the hanging drop methods of vapour diffusion at 20 °C. Psy3-Csm2 crystals were obtained by mixing 1 μl Psy3-Csm2 protein with 1 μl reservoir solution composed of 0.1 M Tris-HCl (pH7.0), 30% Ethylene glycol (in case of Se-Met derivative, 25%) and 5% polyethylene glycol. For cryo-protection, the crystals were transferred into a reservoir solution and the concentration of PEG-400 was increased from 0 to 30%. The crystals were then flash-frozen in cold nitrogen gas stream at 100 K. All X-ray diffraction data were collected at 100 K on the beamlines BL17A of Photon Factory, Tsukuba and BL44XU of SPring-8, Harima, Japan. Native data were obtained at the wavelength of 1.00000 Å. Se-Met derivative data were measures at the wavelength of 0.97888 Å. X-ray diffraction images were processed using the HKL2000 program package [40] . The structure was determined by the single-wavelength anomalous dispersion method using the Se-Met data. Automatic heavy atom location, phasing and phase improvement were performed by solve/resolve [41] at 2.1 Å resolution. The initial model was built by ARP/wARP, then manually built with COOT [42] . The crystallographic refinement was performed by refmac5 (ref. 43 ) at 2.0 Å resolution, and the manual model correction and refinement were iterated until convergence. Geometry of the final model was checked by MolProbity [44] . Statistics of crystallographic analysis is shown in Supplementary Table S1 . All figures showing the atomic structures were drawn with PyMOL(DeLano Scientific, http://www.pymol.org ). Accession code: The structural coordinates for Psy3-Csm2 have been deposited in Protein Data Bank under accession code 3VU9 ; RCSB ID, RCSB095507. How to cite this article: Sasanuma H. et al . A new protein complex promoting the assembly of Rad51 filaments. Nat. Commun. 4:1676 doi: 10.1038/ncomms2678 (2013).